ADAM8 as a drug target in pancreatic cancer Pancreatic ductal adenocarcinoma (PDAC) has a grim prognosis with <5% survivors after 5 years. High expression levels of ADAM8, a metalloprotease disintegrin, are correlated with poor clinical outcome. We show that ADAM8 expression is associated with increased migration and invasiveness of PDAC cells caused by activation of ERK1/2 and higher MMP activities. For biological function, ADAM8 requires multimerization and associates with β1 integrin on the cell surface. A peptidomimetic ADAM8 inhibitor, BK-1361, designed by structural modelling of the disintegrin domain, prevents ADAM8 multimerization. In PDAC cells, BK-1361 affects ADAM8 function leading to reduced invasiveness, and less ERK1/2 and MMP activation. BK-1361 application in mice decreased tumour burden and metastasis of implanted pancreatic tumour cells and provides improved metrics of clinical symptoms and survival in a Kras G12D -driven mouse model of PDAC. Thus, our data integrate ADAM8 in pancreatic cancer signalling and validate ADAM8 as a target for PDAC therapy. Pancreatic ductal adenocarcinoma (PDAC) has the highest mortality rate of solid organ cancers with a 5-year survival rate <5% (ref. 1 ). This cancer type is remarkably homogenous in that 95% of PDAC originate from oncogenic mutations in the KRAS gene. Hence, representative authentic mouse models of PDAC with pancreas-specific expression of Kras have been generated [2] . In mice and man, KRAS mutations cause early-stage pancreatic intraepithelial neoplasias (PanINs) with subsequent development of progressive PDAC. A hallmark of PDAC is the massive infiltration of tumour cells into the pancreas and surrounding tissues including lymphatic organs, spleen and peritoneum, and the concomitant metastasis to the liver and lungs [3] , [4] , [5] , [6] . Infiltration of pancreatic tumour cells depends critically on extracellular matrix (ECM) remodelling [7] , [8] . Given the importance of the ECM in PDAC, the proteolytic release of membrane proteins (shedding) as well as ECM (e.g., collagens and fibronectin) degradation has previously been postulated to have a pivotal role in shaping the tumour microenvironment [9] , [10] . Members of the Metzincin superfamily, matrix metalloproteases (MMPs) and/or ADAM (A disintegrin and metalloproteinase) proteases have been described in these processes [11] . In particular, the contribution of ADAMs to extracellular remodelling [12] and tumour growth, infiltration, metastasis and angiogenesis by shedding of membrane-associated proteins may be important [9] , [13] , [14] . In PDAC patient samples, elevated expression levels of ADAM8 (CD156a, MS2) have been identified versus normal pancreatic tissues. In normal pancreas, ADAM8 expression is very low and restricted to the plasma membrane of ductal cells and, to a lesser extent, of islets and acinar cells. In PDAC tissues, ADAM8 is strongly expressed in tubular complexes and in cancer cells. Based on clinical data, high ADAM8 expression levels are associated with a poor patient prognosis, resulting in reduced survival and increased metastatic spread [15] . ADAM8 is a proteolytically active member of the ADAM protease family originally described in inflammatory processes [16] , [17] , [18] and subsequently in many systems of the body [19] . Increased expression of ADAM8 was observed in other neoplasias, such as high-grade glioma [20] , lung adenocarcinoma [21] , prostate cancer [22] and, more recently, in squamous head and neck cell carcinoma [23] , medulloblastoma [24] , osteosarcoma [25] and breast cancer [26] , suggesting that ADAM8 has an active role in tumour progression. Thus, understanding the functional role of ADAM8 in tumour biology is important. ADAM8 is localized in a few distinct cell types and the analysis of ADAM8-deficient mice inferred dispensability for normal development and homeostasis [27] , [28] . ADAM8 is typically expressed at low levels, giving rise to the current hypothesis that it is functionally irrelevant for homeostasis unless induced by inflammatory stimuli [17] or neoplasias. Once upregulated, ADAM8 can overlap with the substrate spectrum of ADAM10 and ADAM17, two major shedding enzymes, and cleave proteins with immune functions such as tumour necrosis factor receptor 1 (ref. 28 ), L-selectin [29] , CD23 (ref. 30 ) and CXCL1 (ref. 31 ), as well as cell adhesion proteins such as CHL1 (ref. 32 ), thereby potentially modulating immune response or cell adhesion. Cleavage of other ADAM8 substrates such as Tie-2, Flt-1, VE-cadherin, Flk-1, EphB4, KL-1, CD31 and E-selectin [33] or by cleavage of fibronectin [12] may control tumour angiogenesis. Moreover, a role for ADAM8 in metastases [34] and in cell invasiveness [15] , [20] , [22] has been postulated, although the mechanism underlying these processes is unknown. ADAM8 is activated by autocatalysis in the trans-Golgi network [35] and, unlike other ADAMs, not by furine-like convertases. For in vivo activity, ADAM8 requires homophilic multimerization of at least two ADAM8 monomers on the cell membrane. This specific interaction of ADAM8 monomers offers a potential strategy for blocking ADAM8 activity by preventing ADAM8 multimerization in vivo . We have demonstrated previously that ADAM8–ADAM8 interactions critically depend on the disintegrin (DI)/cysteine (DC)-rich domain [35] . In addition, ADAM family members can bind to integrins in vitro via their DC-rich domains [36] ; as prototype, human ADAM15 contains a canonical RGD motif in the integrin-binding loop (IBL) of the DI domain [37] . However, even for non-RGD containing ADAMs such as ADAM9, integrin binding was demonstrated. ADAM9 binding to β1 integrin causes migration of melanoma cells [38] , and for ADAM8, binding to α 9 β 1 was shown in osteoclast turnover [39] , suggesting that these ADAM–integrin interaction have functional relevance. Although ADAM8 has been associated with increased tumour cell migration, invasiveness and metastasis via a combination of catalytic, adhesion and cell signalling functions [15] , [20] , no mechanistic data on ADAM8 in tumour progression and specifically in PDAC are available. Here we provide evidence for an involvement of ADAM8 in cancer signalling and in tumour progression. Furthermore, we validate ADAM8 as a target in PDAC by introducing a specific ADAM8 inhibitor. ADAM8 inhibition strategy Cellular activation of ADAM8 occurs in two steps. The first is intracellular prodomain removal in vesicles, whereas the second is metalloprotease (MP) domain removal from membrane-bound-activated ADAM8 ( Fig. 1a ). Autocatalysis implies that ADAM8 multimerizes ( Fig. 1a ), and that the ADAM8 DC-rich domain is critical for multimerization as demonstrated previously by using an antibody directed against the DC domain [35] . To define the regions in the DC domain involved in ADAM8–ADAM8 interactions, homology modelling of the ADAM8 DC domain was performed based on the ADAM10 sequence derived from Janes et al . [40] ( Supplementary Figs 1 and 2 ). We hypothesized that an extended loop structure exposing the RGD-like positions of the ‘KDX’ motif in the IBL in human and mouse ADAM8 might be responsible for the observed interactions ( Fig. 1b ). 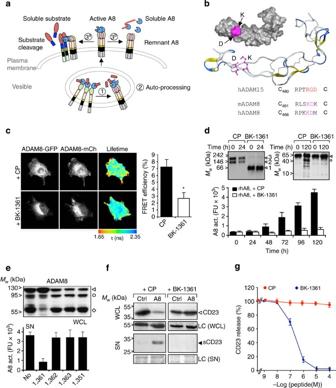Figure 1: Extracellular ADAM8 processing and inhibition of ADAM8 activity. (a) ADAM8 processing: (1) autocatalytic prodomain (red) removal for active ADAM8 (2); after membrane transport, ADAM8 cleaves membrane proteins (3a); alternatively, removal of a soluble MP (blue) domain (3b) leads to ECM cleavage and formation of remnant ADAM8. A putative interaction site (magenta) located in the disintegrin (DI) domain (green). (b) Homology modelling of ADAM8 DC-rich domain based on homology to pdb file 2ao7 (ref.41) within the IBL region of ADAM15. The amino-acid motif ‘KD’ is potentially accessible to peptidomimetics such as BK-1361 (Table 1). (c) FRET analysis of ADAM8 monomers in the presence of BK-1362 (control peptide, CP) and BK-1361 (500 nM) in Panc1 cells. FLIM (in nanoseconds, ns) and FRET efficiency are calculated from >12 cells in three independent experiments. ANOVA was used as statistical test; data are presented as mean±s.e.m.; *P<0.05 (Student’st-test). (d) Left panel, complex of pro-ADAM8 (100 ng per lane) at 0 and 24 h analysed by native gel electrophoresis and immunoblotting. With CP, pro-ADAM8 forms complexes (dimers and trimers, arrowheads 2 and 3); with BK-1361, only monomers of pro-ADMA8 are detected (arrowhead 1); right panel, activation of recombinant pro-ADAM8in vitroin the presence of CP and BK-1361. Bar graph: Autocatalytic activation of pro-ADAM8±BK-1361 (200 nM)in vitro. Pro-ADAM8 (100 ng) incubated for indicated times; Fluorescence activity using CD23 fluorogenic peptide monitored over 5 days in triplicates. FU, fluorescence units. (e) Effect of BK-1361 and CPs (Table 1) on ADAM8 MP domain removal in ADAM8-BiPro-transfected COS7 cells after 12 h. Anti-BiPro antibody detects pro (triangle), mature (circle) and remnant (diamond) ADAM8 in cell lysates (WCLs); soluble ADAM8 activity from processed ADAM8 is detected in cell supernatants (SNs) by CD 23 peptide cleavage. (f) Test of BK-1361 for membrane-bound CD23 in WCLs and soluble CD 23 (sCD23) in SNs. Cells were incubated with CP or BK-1361 (500 nM) for 12 h; ctrl, control; LC, loading control. (g) Dose-dependent inhibition of CD23 shedding determined by ELISA (n=5) with mean values±s.d.; IC50value for BK-1361 was 182±23 nM, whereas CP shows no significant inhibition of CD23 shedding. ADAM8-mCherry, ADAM8-mCh. Figure 1: Extracellular ADAM8 processing and inhibition of ADAM8 activity. ( a ) ADAM8 processing: (1) autocatalytic prodomain (red) removal for active ADAM8 (2); after membrane transport, ADAM8 cleaves membrane proteins (3a); alternatively, removal of a soluble MP (blue) domain (3b) leads to ECM cleavage and formation of remnant ADAM8. A putative interaction site (magenta) located in the disintegrin (DI) domain (green). ( b ) Homology modelling of ADAM8 DC-rich domain based on homology to pdb file 2ao7 (ref. 41 ) within the IBL region of ADAM15. The amino-acid motif ‘KD’ is potentially accessible to peptidomimetics such as BK-1361 ( Table 1 ). ( c ) FRET analysis of ADAM8 monomers in the presence of BK-1362 (control peptide, CP) and BK-1361 (500 nM) in Panc1 cells. FLIM (in nanoseconds, ns) and FRET efficiency are calculated from >12 cells in three independent experiments. ANOVA was used as statistical test; data are presented as mean±s.e.m. ; * P <0.05 (Student’s t -test). ( d ) Left panel, complex of pro-ADAM8 (100 ng per lane) at 0 and 24 h analysed by native gel electrophoresis and immunoblotting. With CP, pro-ADAM8 forms complexes (dimers and trimers, arrowheads 2 and 3); with BK-1361, only monomers of pro-ADMA8 are detected (arrowhead 1); right panel, activation of recombinant pro-ADAM8 in vitro in the presence of CP and BK-1361. Bar graph: Autocatalytic activation of pro-ADAM8±BK-1361 (200 nM) in vitro . Pro-ADAM8 (100 ng) incubated for indicated times; Fluorescence activity using CD23 fluorogenic peptide monitored over 5 days in triplicates. FU, fluorescence units. ( e ) Effect of BK-1361 and CPs ( Table 1 ) on ADAM8 MP domain removal in ADAM8-BiPro-transfected COS7 cells after 12 h. Anti-BiPro antibody detects pro (triangle), mature (circle) and remnant (diamond) ADAM8 in cell lysates (WCLs); soluble ADAM8 activity from processed ADAM8 is detected in cell supernatants (SNs) by CD 23 peptide cleavage. ( f ) Test of BK-1361 for membrane-bound CD23 in WCLs and soluble CD 23 (sCD23) in SNs. Cells were incubated with CP or BK-1361 (500 nM) for 12 h; ctrl, control; LC, loading control. ( g ) Dose-dependent inhibition of CD23 shedding determined by ELISA ( n =5) with mean values±s.d. ; IC 50 value for BK-1361 was 182±23 nM, whereas CP shows no significant inhibition of CD23 shedding. ADAM8-mCherry, ADAM8-mCh. Full size image In mouse and human ADAM8, the amino-acid residues K and D are exposed towards the outer aspect of the DI domain, thereby forming a potential contact interface ( Fig. 1b , labelled in magenta). To generate a peptidomimetic compound, a series of cyclic peptides (six amino acids) mimicking the motif ‘RLSKDK’ of mouse ADAM8 in the IBL were generated. Amino acids R, L or S were inserted in the peptide as D -amino acids to alter the conformational constraint of the KDK motif and to generate a potentially more stable peptide for in vivo work. The cyclic peptide sequence RLsKDK with ‘s’ as D -serine named BK-1361 was most effective in blocking ADAM8-dependent cell adhesion in mouse and human cells with similar efficiencies ( Supplementary Fig. 3 ) and ADAM8–ADAM8 interactions as shown by reduced FRET (Förster resonance energy transfer)/FLIM (fluorescence lifetime imaging) efficiency. In contrast, a control peptide (CP; RLsADK; Fig. 1c ) had no effect. Multimerization of ADAM8 was investigated by native gel electrophoresis ( Fig. 1d ). Under native conditions, 100 ng of pro-ADAM8 associates in dimeric (~120 kDa) and trimeric (~180 kDa) complexes of pro-ADAM8, while in the presence of BK-1361, only monomers (~60 kDa) were detected ( Fig. 1d , left panel). Detection of dimers and trimers suggests that dimers associate by DI domain (homophilic) interactions, whereas trimers could be formed by a different mode of interaction. At higher concentrations of recombinant ADAM8, we detected even larger complexes as a result of greater order multimerization ( Supplementary Fig. 3e ) in agreement with more than one interaction mode that results in ADAM8 complex formation. These interactions can be blocked by BK-1361, and we further analysed whether prevention of complex formation affects ADAM8 activity in vitro. Activation of pro-ADAM8 was detected over a time course of 120 h ( Fig. 1d , right panel) but blocked by BK-1361 ( Fig. 1d , bar graph) with an IC 50 of 120±19 nM. In a cell-based assay, BK-1361 and other peptides ( Table 1 ) were tested for their ability to inhibit ADAM8-dependent extracellular resulting in an active soluble MP domain ( Figs 1a and 3b ). In cell lysates, presence of the remnant form indicates cellular processing of ADAM8 as seen with no or inactive CPs ( Fig. 1e , upper panel). In cell supernatants (SNs), processing results in detectable activity of released ADAM8 MP. BK-1361, but not other BK peptide variants, decreased this activity ( Fig. 1e , lower panel). BK-1361 blocks mouse and human ADAM8 in vitro with similar efficiencies, a prerequisite for testing BK-1361 in orthotopic PDAC models using human donor cells in mouse hosts. Table 1 ADAM8 inhibition by hydroxamates and cyclic peptides. 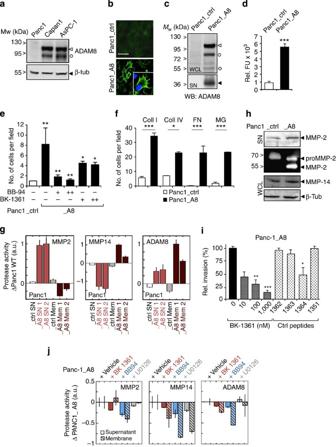Figure 2: Effect of ADAM8 expression in Panc1 cells. (a) Western blotting (WB) of ADAM8 in PDAC cell lines Panc1, Capan-1 and AsPC-1. (b) ADAM8 immunofluorescence (anti-ADAM8, green) in non-permeabilized Panc1_ctrl and Panc1_A8 cells. ADAM8 membrane staining in Panc1_ctrl (upper panel) and Panc1_A8 (lower panel) cells. Insert (lower panel), ADAM8 localization in membrane protrusions. Scale bar, 50 μm. (c) WB of whole-cell lysates (WCLs) and supernatants (SNs) from Panc1_ctrl and Panc1_A8 cells; proform (arrowhead), mature (circle) and remnant form (diamond) of ADAM8, respectively. In Panc1_A8 SN, an ~30-kDa soluble ADAM8 MP fragment is detectable (filled arrowhead). (d) ADAM8 activities in SNs of Panc1_ctrl and Panc1_A8 cells were measured as fluorescence units (FU;n=5) by cleavage of CD23 substrate; ***P<0.0001 (Student’st-test); rel, relative. (e) Scratch assay of Panc1_ctrl versus Panc1_A8 cells treated either with BB-94 (100 nM ‘+’ and 1 μM ‘++’) or with BK-1361 (200 nM ‘+’ and 500 nM ‘++’). Cell counts aftert=0 and 12 h (three independent experiments in triplicates,n=9); ANOVA was used as statistical test; *P<0.01, **P<0.001 (Student’st-test). (f) Invasion of Panc1_ctrl and Panc1_A8 cells in collagen I (Coll I), collagen IV (Coll IV), fibronectin (FN) and Matrigel (MG) analysed in Boyden chambers (18 h). Data are presented as mean±s.d. from five independent experiments. ANOVA test was used. *P<0.01, ***P<0.0001 (Student’st-test). (g) PrAMA inference analysis of SNs and membranes (Mem) from Panc1_ctrl and Panc1_A8 cells using five fluorogenic peptides to detect MMP activities. Activities of MMP-2, MMP-14 and ADAM8 are shown as relative changes to Panc1_ctrl. (h) WB and gelatine zymography of Panc1_ctrl and Panc1_A8 SNs for MMP-2, MMP-2 activity and MMP-14. (i) Invasion of Panc1_A8 cells treated with BK-1361 (10, 100 and 1,000 nM) or 1,000 nM CPs for 6 h (Table 1). Invasion was determined after 18 h. ANOVA test was used. *P<0.005, **P<0.001, ***P<0.0001. (j) PrAMA from Panc1_A8 cells treated with vehicle, BK-1361, BB-94 and U0126 (1 μM, each) for 24 h. Values are given relative to Panc1_A8 treated with vehicle only. ANOVA was used as statistical test. Full size table Figure 2: Effect of ADAM8 expression in Panc1 cells. ( a ) Western blotting (WB) of ADAM8 in PDAC cell lines Panc1, Capan-1 and AsPC-1. ( b ) ADAM8 immunofluorescence (anti-ADAM8, green) in non-permeabilized Panc1_ctrl and Panc1_A8 cells. ADAM8 membrane staining in Panc1_ctrl (upper panel) and Panc1_A8 (lower panel) cells. Insert (lower panel), ADAM8 localization in membrane protrusions. Scale bar, 50 μm. ( c ) WB of whole-cell lysates (WCLs) and supernatants (SNs) from Panc1_ctrl and Panc1_A8 cells; proform (arrowhead), mature (circle) and remnant form (diamond) of ADAM8, respectively. In Panc1_A8 SN, an ~30-kDa soluble ADAM8 MP fragment is detectable (filled arrowhead). ( d ) ADAM8 activities in SNs of Panc1_ctrl and Panc1_A8 cells were measured as fluorescence units (FU; n =5) by cleavage of CD23 substrate; *** P <0.0001 (Student’s t -test); rel, relative. ( e ) Scratch assay of Panc1_ctrl versus Panc1_A8 cells treated either with BB-94 (100 nM ‘+’ and 1 μM ‘++’) or with BK-1361 (200 nM ‘+’ and 500 nM ‘++’). Cell counts after t =0 and 12 h (three independent experiments in triplicates, n =9); ANOVA was used as statistical test; * P <0.01, ** P <0.001 (Student’s t -test). ( f ) Invasion of Panc1_ctrl and Panc1_A8 cells in collagen I (Coll I), collagen IV (Coll IV), fibronectin (FN) and Matrigel (MG) analysed in Boyden chambers (18 h). Data are presented as mean±s.d. from five independent experiments. ANOVA test was used. * P <0.01, *** P <0.0001 (Student’s t -test). ( g ) PrAMA inference analysis of SNs and membranes (Mem) from Panc1_ctrl and Panc1_A8 cells using five fluorogenic peptides to detect MMP activities. Activities of MMP-2, MMP-14 and ADAM8 are shown as relative changes to Panc1_ctrl. ( h ) WB and gelatine zymography of Panc1_ctrl and Panc1_A8 SNs for MMP-2, MMP-2 activity and MMP-14. ( i ) Invasion of Panc1_A8 cells treated with BK-1361 (10, 100 and 1,000 nM) or 1,000 nM CPs for 6 h ( Table 1 ). Invasion was determined after 18 h. ANOVA test was used. * P <0.005, ** P <0.001, *** P <0.0001. ( j ) PrAMA from Panc1_A8 cells treated with vehicle, BK-1361, BB-94 and U0126 (1 μM, each) for 24 h. Values are given relative to Panc1_A8 treated with vehicle only. ANOVA was used as statistical test. 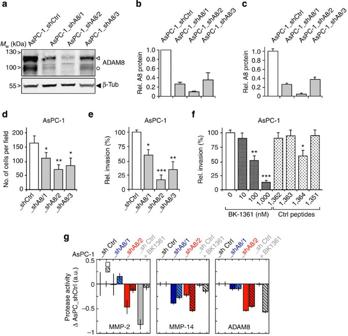Figure 3: ADAM8 inhibition reduces MMP-2 and MMP-14 activity and affects invasiveness. (a) StableADAM8knockdown (shA8) of AsPC-1 cell clones were generated and characterized for ADAM8 protein (b) and mRNA (c) expression; rel, relative. Values are given as mean values from three independent experiments performed in triplicates±s.e.m. Using these cell clones, (d) scratch and (e) Matrigel invasion assays were performed. In both assays, anADAM8gene dosage-dependent effect was observed. (f) Matrigel invasion was determined after addition of BK-1361 (0–1,000 nM) or CPs (Table 1). Ford–f, values are given as mean values±s.e.m. ANOVA was used as statistical test. *P<0.1, **P<0.01, ***P<0.005 (Student’st-test). (g) PrAMA inference analysis of two AsPC-1ADAM8knockdown clones and of AsPC-1_shCtrl cells treated with BK-1361, relative to AsPC-1_shCtrl cells. Note that both genetic and pharmacological inhibition of ADAM8 show similar effects, that is, reduction of MMP-2 and MMP-14 activity with the exception of MMP-14 in AsPC-1 cells. Full size image Figure 3: ADAM8 inhibition reduces MMP-2 and MMP-14 activity and affects invasiveness. ( a ) Stable ADAM8 knockdown (shA8) of AsPC-1 cell clones were generated and characterized for ADAM8 protein ( b ) and mRNA ( c ) expression; rel, relative. Values are given as mean values from three independent experiments performed in triplicates±s.e.m. Using these cell clones, ( d ) scratch and ( e ) Matrigel invasion assays were performed. In both assays, an ADAM8 gene dosage-dependent effect was observed. ( f ) Matrigel invasion was determined after addition of BK-1361 (0–1,000 nM) or CPs ( Table 1 ). For d – f , values are given as mean values±s.e.m. ANOVA was used as statistical test. * P <0.1, ** P <0.01, *** P <0.005 (Student’s t -test). ( g ) PrAMA inference analysis of two AsPC-1 ADAM8 knockdown clones and of AsPC-1_shCtrl cells treated with BK-1361, relative to AsPC-1_shCtrl cells. Note that both genetic and pharmacological inhibition of ADAM8 show similar effects, that is, reduction of MMP-2 and MMP-14 activity with the exception of MMP-14 in AsPC-1 cells. Full size image We next tested BK-1361 and variants for their ability to inhibit shedding of CD23, a known substrate of ADAM8 (ref. 30 ) in cell-based shedding assays ( Fig. 1f and Table 1 ). Co-transfection of ADAM8 with a tagged CD23 construct in COS7 cells resulted in significant shedding of CD23 as soluble 21 kDa fragment (sCD23); sCD23 was detectable in SNs when ADAM8 was co-expressed. In the presence of 500 nM BK-1361, sCD23 was undetectable, demonstrating that BK-1361 inhibits the in vivo shedding activity of ADAM8. Enzyme-linked immunosorbent assay (ELISA) assays were performed to determine [sCD23] versus [BK-1361] with an IC 50 of 182±23 nM for BK-1361; BK-1362 had no significant effect ( Fig. 1g ). We conclude that BK-1361 affects ADAM8–ADAM8 interactions, thereby inhibiting cellular shedding and autocatalytic activation of ADAM8 in vitro and in a cell-based assay in a specific manner, as neither catalytic activities of ADAM9, -10, -12 and -17 nor MMP-2, -9 and -14 were inhibited in concentrations of up to 10 μM ( Table 2 ). Table 2 Specificity of BK-1361 against other ADAM proteases and MMPs. Full size table ADAM8 induces migration/invasion of pancreatic cancer cells As shown earlier, ADAM8 expression is correlated with invasiveness in vitro in various cell lines [15] , [20] , [21] . However, no functional in vivo data on ADAM8 in pancreatic malignancies are yet available. To establish cell lines for analysis of PDAC in vivo , we selected Panc1 (very low ADAM8) and AsPC-1 cells (high endogenous levels of ADAM8) as determined by western blotting [15] ( Fig. 2a ). Panc1 cell lines with a moderate overexpression of ADAM8 (Panc1_A8; NM_001109.4; Fig. 2b ) and AsPC-1 cell lines with ADAM8 shRNA knockdown constructs were generated. Microarray analysis of Panc1_ctrl versus Panc1_A8 cells revealed that Panc1_A8 cells showed no off-target effects of the ADAM8 knockdown, as expression levels of >95% of genes were unchanged, including genes encoding MMPs, other ADAMs, ADAMTS and TIMP1–4 levels ( Supplementary Fig. 4 ). Cellular localization of ADAM8, analysed by confocal laser-scanning microscopy, confirmed low ADAM8 expression in Panc1_ctrl cells compared with enhanced ADAM8 expression in Panc1_A8 cells. In Panc1_A8 cells, ADAM8 is localized in the cell membrane and membrane extrusions ( Fig. 2b ). In SNs of different Panc1_A8 cell clones characterized ( n =30), ADAM8 catalytic activity correlated with the ADAM8 dosage, determined by western blotting ( Fig. 2c ) and CD23 fluorescence assay ( Fig. 2d ). Migration and invasion behaviour of Panc1_ctrl cells was compared with Panc1_A8 cells in vitro ( Fig. 2e,f ). In wound-healing (scratch) assays, migration rates of Panc1_A8 cells were significantly increased (8±3.8-fold) compared with Panc1_ctrl cells. Panc1_A8 cell migration is inhibited by BB-94, a MP inhibitor. In addition, application of BK-1361 reduced migration rates of Panc1_A8 cells significantly, but not to the same level as BB-94, suggesting that ADAM8 modulates other MP activities accounting for migration above control levels. Accordingly, invasion into different ECM substrates such as collagen I, collagen IV, fibronectin and Matrigel was enhanced by ADAM8 ( Fig. 2f ). ADAM8 increases extracellular MMP activity A proteolytic activity matrix assay (PrAMA) [41] was used for simultaneous detection of multiple activities in Panc1_ctrl and Panc1_A8 cells that could account for the observed invasiveness. Briefly, PrAMA is based on the knowledge of individual FRET-substrate MMP/ADAM cleavage signatures using purified enzymes [41] . Panels of FRET-substrate cleavage measurements can be used to infer a dynamic, quantitative and specific profile of MMP/ADAM proteolytic activities from complex enzyme mixtures such a SNs and solubilized membranes (see Methods and Supplementary Fig. 5 ). PrAMA inference revealed increased activities of MMP-2 in SNs and MMP-14 (MT1-MMP) in cell membranes of Panc1_A8 cells compared with Panc1_ctrl cells ( Fig. 2g and Supplementary Fig. 5 ). Enhanced ADAM8 activities were detected in SNs and membranes of Panc1_A8 cells. Gelatine zymography and western blotting for MMP-2 and MMP-14 confirmed increased activity of MMP-2 and higher membrane concentration of MT1-MMP ( Fig. 2h ). However, elevated MMP activities in Panc1_A8 cells are not due to transcriptional activation of MMP-2 and MMP-14 ( Supplementary Fig. 4 ). We further investigated whether BK-1361 is able to affect ADAM8-dependent invasiveness and MMP secretion of Panc1_A8 cells ( Fig. 2i,j ). BK-1361 and peptide variants were tested for their ability to block invasiveness of Panc1_A8 cells ( Fig. 2i ). A dose-dependent effect of BK-1361 on invasion of Panc1_A8 cells was observed. From CPs, only BK-1364 had a slight effect on invasion. In parallel, we performed PrAMA assays in Panc1_A8 cells to evaluate MMP-2, MMP-14, and ADAM8 activities in the presence of BK-1361, BB-94 and the extracellular regulated kinase (ERK) inhibitor U0126, respectively ( Fig. 2j ). BK-1361 and BB-94 reduced activities of MMP-2, MMP-14 and ADAM8. ERK inhibition had a slight effect on MMP-2 activity and a greater effect on MMP-14 activity, whereas ADAM8 activity was not affected. These findings argue for an ERK1/2-mediated effect on MMP-14, and, to a lesser extent, on MMP-2 activation. ADAM8 as regulator of ERK1/2 activation is not directly affected by U0126. Our data suggest an effect of pharmacological ADAM8 inhibition on invasiveness of PDAC cells. To determine the effect of a genetic ADAM8 knockdown on cellular invasiveness, we selected AsPC-1 cells with high endogenous ADAM8 levels ( Fig. 2a ) and generated AsPC_1 cell clones carrying a stable knockdown of ADAM8 (sh_A8). Three representative cell clones from different sh_A8 constructs were analysed for ADAM8 expression ( Fig. 3a–c ), cell migration and invasion ( Fig. 3d,e and Supplementary Movies 1, 2 ). Knockdown of ADAM8 in AsPC-1 cells caused a significant drop in cell migration depending on the gene dosage of ADAM8. Invasion of AsPC-1 cells was similarly affected by ADAM8 dosage ( Fig. 3e ). BK-1361 treatment of wild-type (wt) AsPC-1 cells was similar to the genetic knockdown of ADAM8 with 87±3.5% inhibition ( Fig. 3f ). PrAMA assays were performed with AsPC-1_shCtrl±BK-1361 and AsPC-1_shA8 cell clones 1 and 2 ( Fig. 3g ). Reduction of MMP-2 and MMP-14 activities were observed in AsPC-1_shA8 clones. In BK-1361-treated AsPC-1_shCtrl cells, MMP-2 was similarly affected, however, the effect on MMP-14 was less pronounced ( Fig. 3g ). ADAM8 interacts with integrin β1 in pancreatic cancer cells The membrane localization of ADAM8 in Panc1_A8 cells suggests that ADAM8 is complexed with cellular integrins, thereby enhancing cell migration and invasiveness. To investigate this, co-immunoprecipitation (co-IP) experiments were performed in Panc1 cells expressing either control or a tagged ADAM8 construct (ADAM8-BiPro). As a result, β1 integrin, present in comparable amounts in Panc1_ctrl and Panc1_A8 cells, was co-IP with ADAM8 ( Fig. 4a–c ). To analyse cellular ADAM8-β1 integrin and ADAM8–ADAM8 interactions, FRET/FLIM analyses were performed to detect FRET in cell lines expressing fusion proteins ADAM8-GFP and ADAM8-mCherry, respectively. ADAM8 multimerization was detected in Panc1 cells ( Fig. 4d,e ), indicated by FRET efficiency of 7.5±0.93%. In cells, complex formation and membrane localization of ADAM8 in vivo involves β1 integrin, since treatment of Panc1 cells with a β1 integrin-blocking antibody ( Fig. 4d,e ) resulted in a significant drop to 3.1±0.8% FRET efficiency. Moreover, MDA-MB-231 breast cancer cells lacking β1 integrin ( Fig. 4f,g ) show a significant change in cellular morphology while ADAM8 localization in lamellipod structures is lost. Interestingly, administration of BK-1361 causes a similar change in cell morphology ( Fig. 4h,i ). We conclude that β1 integrin knockdown or specific ADAM8 inhibition have similar effects on ADAM8 membrane localization ( Fig. 4j ). In addition, areas of positive ADAM8-FRET in MDA-MB-231 cells were analysed for β1 integrin ( Fig. 4k,l ). In most areas, activated β1 integrin was detected by antibody 12G10, suggesting that ADAM8 interaction and β1 integrin activation are correlated. 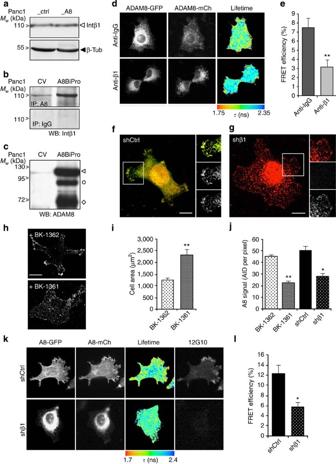Figure 4: ADAM8 multimerizes and interacts with integrin β1 in tumour cells. (a) Western blot (WB) of integrin β1 subunit (Int β1) in Panc1_ctrl (ctrl) and Panc1_A8 (A8) cells (~115 kDa). β-Tubulin (β-tub) was used as loading control. (b) In Panc1 cells transiently expressing control vector (CV) or ADAM8-Bipro (A8BiPro), anti-BiPro or unrelated IgG was used for immunoprecipitation (IP). Blots were probed with polyclonal β1 integrin antibody. (c) Re-probing of blot (b) using polyclonal anti-ADAM8 antibody. (d) FRET/FLIM analysis of ADAM8–ADAM8 interactions. Panc1 cells were co-transfected with ADAM8-GFP and ADAM8-mCherry (A8-mCh) constructs; (upper panel) FLIM in the absence (control IgG) and (lower panel) in the presence of anti-β1 antibody (anti-β1), determined in nanoseconds (ns). (e) FRET efficiency (in %) for ADAM8–ADAM8 interaction in anti-β1 antibody-treated Panc1 cells (n=10). As statistical test, ANOVA was used; **P<0.001. (f–h) Localization of ADAM8 protein in MDA-MB-231 control (shCtrl,f) or (h) in MDA-MB-231 cells with a stable β1 integrin knockdown. Staining of ADAM8 in red and β1 integrin in green. Boxed areas infare a lamellipod structure zoomed in. In contrast to boxed area inf, the one ingshows diffuse staining of ADAM8 mainly in vesicles, the entire cell is flattened and cell area increases significantly. Scale bars (f,g), 10 μm. (h) Localization of ADAM8 in MDA-MB-231 cells treated with peptide BK-1362 (1μM) or with BK-1361 (1μM). Similar tog, cells flatten and localization of ADAM8 in lamellipodia is changed. (i) Quantification of cell areas of BK-1362- and BK-1361-treated cells, given as mean ±s.d. from 50 cell areas. **P<0.001 (Student’st-test). (j) Quantification of ADAM8 in the cell membrane as average integrated density (AID) per pixel (sum of density 5 μm in from cell periphery, divided by total pixels). ANOVA was used as statistical test. *P<0.01, **P<0.001 (Student’st-test). (k) Interaction of ADAM8-GFP and ADAM8-mCh in MDA-MB-231 control (shCtrl) and MDA-MB-231 with a stable β1 integrin knockdown (shβ1). In the right panel, antibody 12G10 was used to detect activated β1 integrin. (l) Quantification of FRET efficiency between ADAM8-GFP and ADAM8-mCh in MDA-MB-231 control (shCtrl) and MDA-MB-231 with stable β1 integrin knockdown (shβ1). ANOVA was used; *P<0.01 and **P<0.001 (Student’st-test). Figure 4: ADAM8 multimerizes and interacts with integrin β1 in tumour cells. ( a ) Western blot (WB) of integrin β1 subunit (Int β1) in Panc1_ctrl (ctrl) and Panc1_A8 (A8) cells (~115 kDa). β-Tubulin (β-tub) was used as loading control. ( b ) In Panc1 cells transiently expressing control vector (CV) or ADAM8-Bipro (A8BiPro), anti-BiPro or unrelated IgG was used for immunoprecipitation (IP). Blots were probed with polyclonal β1 integrin antibody. ( c ) Re-probing of blot ( b ) using polyclonal anti-ADAM8 antibody. ( d ) FRET/FLIM analysis of ADAM8–ADAM8 interactions. Panc1 cells were co-transfected with ADAM8-GFP and ADAM8-mCherry (A8-mCh) constructs; (upper panel) FLIM in the absence (control IgG) and (lower panel) in the presence of anti-β1 antibody (anti-β1), determined in nanoseconds (ns). ( e ) FRET efficiency (in %) for ADAM8–ADAM8 interaction in anti-β1 antibody-treated Panc1 cells ( n =10). As statistical test, ANOVA was used; ** P <0.001. ( f – h ) Localization of ADAM8 protein in MDA-MB-231 control (shCtrl, f ) or ( h ) in MDA-MB-231 cells with a stable β1 integrin knockdown. Staining of ADAM8 in red and β1 integrin in green. Boxed areas in f are a lamellipod structure zoomed in. In contrast to boxed area in f , the one in g shows diffuse staining of ADAM8 mainly in vesicles, the entire cell is flattened and cell area increases significantly. Scale bars ( f , g ), 10 μm. ( h ) Localization of ADAM8 in MDA-MB-231 cells treated with peptide BK-1362 (1μM) or with BK-1361 (1μM). Similar to g , cells flatten and localization of ADAM8 in lamellipodia is changed. ( i ) Quantification of cell areas of BK-1362- and BK-1361-treated cells, given as mean ±s.d. from 50 cell areas. ** P <0.001 (Student’s t -test). ( j ) Quantification of ADAM8 in the cell membrane as average integrated density (AID) per pixel (sum of density 5 μm in from cell periphery, divided by total pixels). ANOVA was used as statistical test. * P <0.01, ** P <0.001 (Student’s t -test). ( k ) Interaction of ADAM8-GFP and ADAM8-mCh in MDA-MB-231 control (shCtrl) and MDA-MB-231 with a stable β1 integrin knockdown (shβ1). In the right panel, antibody 12G10 was used to detect activated β1 integrin. ( l ) Quantification of FRET efficiency between ADAM8-GFP and ADAM8-mCh in MDA-MB-231 control (shCtrl) and MDA-MB-231 with stable β1 integrin knockdown (shβ1). ANOVA was used; * P <0.01 and ** P <0.001 (Student’s t -test). Full size image To analyse whether ADAM8 interactions cause altered intracellular signalling, a mitogen-activated protein kinase (MAPK) array was used to screen for kinase phosphorylation in Panc1_ctrl and Panc1_A8 cells ( Supplementary Fig. 6 ). As potential downstream effectors of the observed ADAM8-β1 integrin interaction, we investigated phosphorylation of focal adhesion kinase (FAK), ERK1/2, Akt and p38 γ in Panc1_A8 versus Panc1_ctrl cells. Focal adhesion kinase was described as β1 integrin interacting protein [42] . In western blots, increased phosphorylation of FAK at residue Tyr397 correlates with ADAM8 expression levels in Panc1 cells ( Fig. 5a ). In addition to pFAK, we detected increased phosphorylation of ERK1/2 (p44/p42) in Panc1_A8 cells by western blotting using corresponding phospho-specific antibodies (3.4-fold±0.2 Panc1_A8 versus Panc1_ctrl; Fig. 5b ). The observed increase in pERK1/2 was reduced in Panc1_A8 cells treated with BK-1361 ( Fig. 5b ). To correlate ERK1/2 phosphorylation with the observed invasiveness of Panc1 cells, Matrigel invasion assays were performed in the presence of U0126 ( Fig. 5c ). U0126 blocked ERK1/2 phosphorylation in Panc1_ctrl and Panc1_A8 cells, and resulted in decreased invasion of Panc1_A8 cells. In addition, AsPC-1_shCtrl and three AsPC-1_shA8 cell clones with different ADAM8 levels were analysed for pERK1/2 levels ( Fig. 5d ). In cell clone AsPC-1_shA8/2, pERK1/2 levels were reduced by 2.9±0.3 fold, suggesting that ADAM8 expression levels are correlated with pERK1/2. In AsPC-1 cells, ADAM8 levels affect MEK1/2, p-Akt and c-Raf activation ( Fig. 5e ). In addition, a β1 integrin antibody that blocks activation was able to reduce pERK1/2 levels in Panc1_A8 cells, demonstrating that β1 integrin is required for ADAM8-dependent ERK1/2 activation ( Supplementary Fig. 7 ). 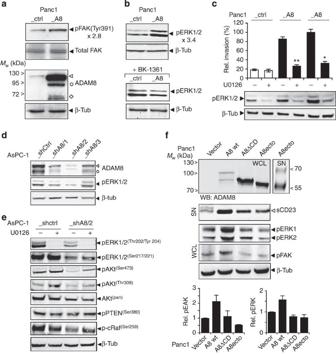Figure 5: ADAM8 intracellular kinase signalling. (a) Antibody detection of FAK phosphorylation (Y397) in Panc1_A8 and Panc1_ctrl cells 24 h after plating cells on plastic. Total FAK antibody was used to control equal loading and anti-ADAM8 confirms ADAM8 expression. A β-tubulin antibody was used as loading control. Note a 2.8-fold increase in pFAK in Panc1_A8 cells compared with Panc1_ctrl cells. (b) Western blotting (WB) of relative (rel.) phosphorylation of ERK1/2, in Panc1_ctrl and Panc1_A8 cells as determined by antibodies directed against phosphorylated forms of respective kinases. Lower panel, ERK1/2 phosphorylation in Panc1_ctrl and Panc1_A8 cells in the presence of 500 nM BK-1361. (c) Relative invasiveness of Panc1_ctrl and Panc1_A8 cells (in duplicates) in the presence of ERK1/2 inhibitor U0126 (10 μM) after 18 h incubation, indicating a strong correlation between ERK1/2 phosphorylation and invasion in Panc1 cells. ANOVA statistical test was used; *P<0.01, **P<0.001 (Student’st-test). (d) Correlation of ADAM8 and pERK1/2 levels in AsPC-1 control (shCtrl) and knockdown (shA8) cells. In clone AsPC-1_shA8/2, levels of pERK1/2 are reduced by threefold. (e) Relative kinase phosphorylation of the ERK and AKT signalling pathways after 18 h incubation with (+) or without (−) U0126 (10 μM) in protein lysates of AsPC-1_shCtrl and AsPC-1_shA8 cells. Kinases and their respective phosphorylation sites are indicated on the right. (f) Membrane-bound ADAM8 with cytoplasmic domain is required for FAK and ERK1/2 activation. Panc1 cells were transiently transfected with full-length ADAM8 construct (A8 wt), ADAM8 lacking the cytoplasmic domain (A8ΔCD), or with a construct encoding the soluble ectodomain (A8ecto) of ADAM8, respectively. To control for cellular ADAM8 activity, the amount of soluble CD23 was determined in SNs by using an HA-tag antibody. The presence of ADAM8 protein variants, relative levels of pFAK and pERK1/2 were detected by WB, using β-tubulin as loading control. Levels of FAK and ERK phosphorylation were quantified from three independent experiments, given as mean±s.e.m. WCL, whole-cell lysates. Figure 5: ADAM8 intracellular kinase signalling. ( a ) Antibody detection of FAK phosphorylation (Y397) in Panc1_A8 and Panc1_ctrl cells 24 h after plating cells on plastic. Total FAK antibody was used to control equal loading and anti-ADAM8 confirms ADAM8 expression. A β-tubulin antibody was used as loading control. Note a 2.8-fold increase in pFAK in Panc1_A8 cells compared with Panc1_ctrl cells. ( b ) Western blotting (WB) of relative (rel.) phosphorylation of ERK1/2, in Panc1_ctrl and Panc1_A8 cells as determined by antibodies directed against phosphorylated forms of respective kinases. Lower panel, ERK1/2 phosphorylation in Panc1_ctrl and Panc1_A8 cells in the presence of 500 nM BK-1361. ( c ) Relative invasiveness of Panc1_ctrl and Panc1_A8 cells (in duplicates) in the presence of ERK1/2 inhibitor U0126 (10 μM) after 18 h incubation, indicating a strong correlation between ERK1/2 phosphorylation and invasion in Panc1 cells. ANOVA statistical test was used; * P <0.01, ** P <0.001 (Student’s t -test). ( d ) Correlation of ADAM8 and pERK1/2 levels in AsPC-1 control (shCtrl) and knockdown (shA8) cells. In clone AsPC-1_shA8/2, levels of pERK1/2 are reduced by threefold. ( e ) Relative kinase phosphorylation of the ERK and AKT signalling pathways after 18 h incubation with (+) or without (−) U0126 (10 μM) in protein lysates of AsPC-1_shCtrl and AsPC-1_shA8 cells. Kinases and their respective phosphorylation sites are indicated on the right. ( f ) Membrane-bound ADAM8 with cytoplasmic domain is required for FAK and ERK1/2 activation. Panc1 cells were transiently transfected with full-length ADAM8 construct (A8 wt), ADAM8 lacking the cytoplasmic domain (A8ΔCD), or with a construct encoding the soluble ectodomain (A8ecto) of ADAM8, respectively. To control for cellular ADAM8 activity, the amount of soluble CD23 was determined in SNs by using an HA-tag antibody. The presence of ADAM8 protein variants, relative levels of pFAK and pERK1/2 were detected by WB, using β-tubulin as loading control. Levels of FAK and ERK phosphorylation were quantified from three independent experiments, given as mean±s.e.m. WCL, whole-cell lysates. Full size image To investigate whether the observed FAK and ERK1/2 activation depends on membrane-bound ADAM8, Panc1 cells were transfected with wt ADAM8 (A8 wt), an ADAM8 construct lacking the cytoplasmic domain (A8ΔCD), or a soluble ADAM8 (A8ecto) construct ( Fig. 5f ). First, we confirmed that all constructs are catalytically active, as all three ADAM8 proteins shed CD23 (sCD23) from the cell membrane. Interestingly, neither ΔCD nor the ectodomain of ADAM8 were able to activate FAK and ERK1/2 ( Fig. 5f ), suggesting that intracellular signalling mediated by ADAM8 requires membrane localization of ADAM8 and the presence of the cytoplasmic domain. As potential substrates for ERK activation, that is, the epidermal growth factor receptor (EGFR) ligand family such as Heparin-binding epidermal growth factor (HB-EGF), EGF or amphiregulin, were screened ( Supplementary Fig. 8 ). We have not identified significant EGFR ligand release, so that ADAM8–β1 integrin interactions might act independent from EGFR signalling. Role of ADAM8 in PDAC and effect of BK-1361 in vivo Based on our findings that ADAM8 inhibition blocks invasiveness and ERK1/2 signalling in PDAC cells, we used BK-1361 to validate ADAM8 as a therapeutic target in PDAC in vivo . Initially, acute and chronic toxicity analyses were performed in C57BL/6J mice. In single and repeated dose applications, doses of up to 10 μg g −1 body weight were well tolerated as mice showed no abnormalities, weight loss or motor performance over 4 weeks. After necropsy, organs investigated showed no abnormalities at histological level ( Supplementary Fig. 9 ). Owing to the lack of acute and chronic toxicity, a dose of 10 μg g −1 body weight was applied daily for subsequent in vivo applications. Initially, orthotopic injections of Panc1 cells into mouse pancreas were performed ( Fig. 6a–g ) in three cohorts ( n =12 each); cohort 1 received Panc1_A8 cells, cohort 2 received Panc1_ctrl cells and cohort 3 received Panc1_A8 cells followed by daily intraperitoneal injection of 10 μg g −1 BK-1361. Mice were monitored for 12 days, by which time most of the mice injected with Panc1_A8 cells were moribund and reached end point criteria. In contrast, mice injected with Panc1_ctrl cells or Panc1_A8/BK-1361 treatment showed improved clinical parameters. At end point, pancreatic tumours formed from Panc1_ctrl cells were significantly smaller than from Panc1_A8 cells ( Fig. 6a,b ). Moreover, tumours obtained from mice that received Panc1_A8 cells and daily injections of BK-1361 were significantly smaller. These data indicate that inhibition of ADAM8 reduced tumour load to almost the value of Panc1_ctrl-derived tumours (0.42 g for Panc1_ctrl versus 0.62 g for Panc1_A8/BK-1361). By histology, a significant invasion of Panc1_A8 cells into the pancreatic tissue was detected, whereas in tumours derived from Panc1_A8/BK-1361 cells, tumour masses embedded in Matrigel were primarily localized to the implantation site even after 12 days, as the boundaries of pancreas and implanted tumour mass were still distinct ( Fig. 6c ). In addition, there were signs of necrosis inside the implanted tumour treated with BK-1361 ( Fig. 6c ), inferring that non-invasive Panc1 cells undergo necrotic changes. Moreover, ADAM8 levels in Panc1_ctrl cells located in the tumour were increased under hypoxic conditions. Co-staining for pERK1/2 was observed in infiltrative ADAM8-positive tumour cells ( Fig. 6d , upper panel). 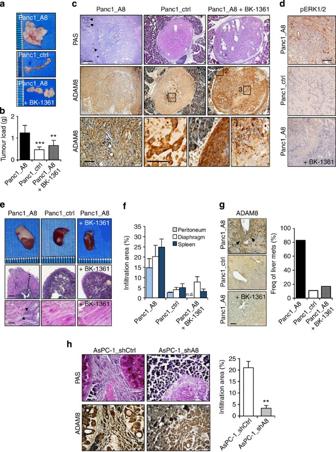Figure 6: Effect of ADAM8 inhibition in an orthotopic pancreatic cancer model. (a) Pancreas morphology after orthotopic injection of Panc1_A8, Panc1_ctrl or Panc1_A8 cells followed by BK-1361 injection (10 μg g−1daily,n=12 per group). (b) Tumour load (g) 12 days after implantation (n=12); Tukey’s linear contrast test was used. **P<0.001, ***P<0.0001 (Student’st-test) (c) Representative ADAM8 IHC/Periodic Acid Schiffs (PAS) staining of pancreas tumours from mice injected with Panc1_A8, Panc1_ctrl compared with implanted Panc1_A8/BK-1361 treated. Significant invasion of Panc1_A8 cells (arrows, upper panel left); across the implantation border (asterisk, upper left panel); Panc1_ctrl and Panc1_A8/BK-1361 injected tumours show less invasion from implantation site. Lower panel, ADAM8 staining; infiltration and loss of ductal architecture, increase in ADAM8 in Panc1_ctrl-implanted tumours and delineated between implantation site and surrounding pancreas tissue in Panc1_A8/BK-1361-treated mice. Lower left panel, enlarged image shows invasion of ADAM8-positive tumour cells; enlarged images (boxed in upper panel); box1: upregulation of ADAM8 in cell mass of Panc1_ctrl cells; box 2: enlarged view of the border between implantation site and surrounding ductal tissue; box 3: signs of intratumoral necrosis in tumours treated with BK-1361 (scale bars, 100 μm). (d) pERK1/2 staining of tumours. Only for Panc1_A8 (top), tumour cells stain positive for pERK1/2 (scale bar, 100 μm). (e) Morphology of spleen and diaphragm from mice injected with either Panc1_A8, Panc1_ctrl, or Panc1_A8/BK-1361. In PAS stains (lower panel), infiltration of tumour cells in the diaphragm is only seen in Panc1_A8. Scale bars, 100 μm. (f) Quantification of infiltration areas in peritoneum, diaphragm and spleen. Values are in % of total tissue area ±s.e.m. (n=12). (g) ADAM8+micrometastases in livers from Panc1_A8-injected mice; in contrast, metastases (mets) were mostly absent in livers from Panc1_ctrl and Panc1_A8/BK-1361-treated mice (scale bar, 200 μm); relative frequency (Freq.) of liver metastases in mice injected with Panc1_A8, Panc1_ctrl and Panc1_A8/BK-1361, respectively (n=12). (h) Pancreas histology (PAS, ADAM8 IHC) after orthotopic implantation of AsPC-1_shCtrl and AsPC-1_shA8/2 cells. Scale bar, left upper panel, 100 μm. ADAM8+cells in pancreas injected with AsPC-1_shCtrl cells, weaker staining with AsPC-1_shA8 cells. Infiltration areas in pancreata from six mice per group were quantified. Mean±s.e.m. **P<0.01 (Student’st-test). Figure 6: Effect of ADAM8 inhibition in an orthotopic pancreatic cancer model. ( a ) Pancreas morphology after orthotopic injection of Panc1_A8, Panc1_ctrl or Panc1_A8 cells followed by BK-1361 injection (10 μg g −1 daily, n =12 per group). ( b ) Tumour load (g) 12 days after implantation ( n =12); Tukey’s linear contrast test was used. ** P <0.001, *** P <0.0001 (Student’s t -test) ( c ) Representative ADAM8 IHC/Periodic Acid Schiffs (PAS) staining of pancreas tumours from mice injected with Panc1_A8, Panc1_ctrl compared with implanted Panc1_A8/BK-1361 treated. Significant invasion of Panc1_A8 cells (arrows, upper panel left); across the implantation border (asterisk, upper left panel); Panc1_ctrl and Panc1_A8/BK-1361 injected tumours show less invasion from implantation site. Lower panel, ADAM8 staining; infiltration and loss of ductal architecture, increase in ADAM8 in Panc1_ctrl-implanted tumours and delineated between implantation site and surrounding pancreas tissue in Panc1_A8/BK-1361-treated mice. Lower left panel, enlarged image shows invasion of ADAM8-positive tumour cells; enlarged images (boxed in upper panel); box1: upregulation of ADAM8 in cell mass of Panc1_ctrl cells; box 2: enlarged view of the border between implantation site and surrounding ductal tissue; box 3: signs of intratumoral necrosis in tumours treated with BK-1361 (scale bars, 100 μm). ( d ) pERK1/2 staining of tumours. Only for Panc1_A8 (top), tumour cells stain positive for pERK1/2 (scale bar, 100 μm). ( e ) Morphology of spleen and diaphragm from mice injected with either Panc1_A8, Panc1_ctrl, or Panc1_A8/BK-1361. In PAS stains (lower panel), infiltration of tumour cells in the diaphragm is only seen in Panc1_A8. Scale bars, 100 μm. ( f ) Quantification of infiltration areas in peritoneum, diaphragm and spleen. Values are in % of total tissue area ±s.e.m. ( n =12). ( g ) ADAM8 + micrometastases in livers from Panc1_A8-injected mice; in contrast, metastases (mets) were mostly absent in livers from Panc1_ctrl and Panc1_A8/BK-1361-treated mice (scale bar, 200 μm); relative frequency (Freq.) of liver metastases in mice injected with Panc1_A8, Panc1_ctrl and Panc1_A8/BK-1361, respectively ( n =12). ( h ) Pancreas histology (PAS, ADAM8 IHC) after orthotopic implantation of AsPC-1_shCtrl and AsPC-1_shA8/2 cells. Scale bar, left upper panel, 100 μm. ADAM8 + cells in pancreas injected with AsPC-1_shCtrl cells, weaker staining with AsPC-1_shA8 cells. Infiltration areas in pancreata from six mice per group were quantified. Mean±s.e.m. ** P <0.01 (Student’s t -test). Full size image Metastasis and infiltration is the major cause for the observed morbidity in PDAC [5] , [6] . Since ADAM8 was discussed in the context of infiltration and metastasis [26] , [34] , we investigated orthotopic mice for infiltration of close structures such as peritoneum, diaphragm and spleen, and liver metastasis. From mice injected with Panc1_A8 cells, we found significant infiltrates in adjacent organs ( Fig. 6e,f ). Macroscopic inspection and haematoxylin/eosin stain of tissue sections revealed higher invasion into spleen and diaphragm of Panc1_A8-injected mice ( Fig. 6e ). Analysis of infiltration areas showed enhanced invasive behaviour of Panc1_A8 cells versus Panc1_ctrl and Panc1_A8/BK-1361 cells ( Fig. 6f ) in peritoneum, diaphragm and spleen. ADAM8 staining of liver sections revealed occurrence of micrometastases with higher frequencies in Panc1_A8 implanted mice compared with Panc1_ctrl and Panc1_A8/BK-1361 ( Fig. 6g ). Metastases frequencies were markedly different between Panc1_A8, Panc1_ctrl and Panc1_A8/BK-1361. Furthermore, the implantation of AsPC-1_shCtrl and AsPC-1_shA8 cells was analysed ( Fig. 6h ). AsPC-1_shCtrl cells caused large streams of tumour cells invading the pancreatic tissue with an infiltration area of 21±2.8%. In contrast, AsPC-1_shA8 cells were located close to the injection site and showed less invasive behaviour with infiltration areas of 3.4±1.2% ( P <0.01). Thus, data derived from genetic ADAM8 knockdown support the results obtained with ADAM8 inhibition using BK-1361. The therapeutic effect of ADAM8 inhibition in vivo was analysed in mice with genotype Kras LSL-G12D , Trp53 R172H/+ , Pdx Cre/+ (KPC) [2] , a genetically engineered PDAC mouse model. Injections of BK-1361 were started around the onset of PanINs. KPC control groups received injections of either saline (as in a clinical setting) or CP (BK-1362). Control groups showed progression to PDAC with a median survival of 15.5 weeks for saline and 16 weeks for BK-1362. In contrast, BK-1361-treated KPC mice have extended median survival times of 24.2 weeks ( Fig. 7a ). The in vivo efficacy of BK-1361 was demonstrated by determining soluble ADAM8 levels ( Fig. 7b ). Lower frequencies of metastases in liver and lung were observed in BK-1361-treated KPC mice ( Fig. 7c ). Pancreas morphology in BK-1361-treated mice showed reduced infiltration areas in the pancreas compared with control mice ( Fig. 7d,e ), while the areas of intact acinar structures are increased (0.74% for BK-1361-treated versus 0.18% for saline-treated mice, Fig. 7f ). Tumour progression was associated with increased staining for ADAM8 and pERK1/2 in control KPC mice. In BK-1361-treated KPC mice, ADAM8 and pERK1/2 staining is restricted to acinar structures, suggesting that despite occurrence of neoplasias, tumour infiltration was reduced while the acinar architecture was more conserved ( Fig. 7g ). Staining intensities of pERK1/2 and ADAM8 is reduced in BK-1361-treated KPC mice ( Fig. 7h ), suggesting that, in vivo , ADAM8 inhibition leads to reduced activation of pERK1/2. 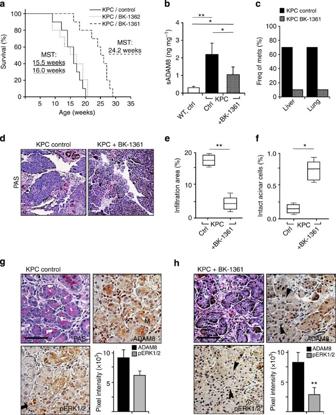Figure 7: Application of peptide BK-1361 in PDAC mice. (a) Kaplan–Meier analysis of KPC/saline, KPC/BK-1362 (CP) and KPC/BK-1361 mice (n=10 in each group). Median survival times (MSTs) are given in the diagram; statistical analysis was carried out using a log-rank test withP<0.001. (b) Concentration of soluble ADAM8 (sADAM8) in normal mouse pancreas (wt) and in pancreata of saline-treated and BK-1361-treated KPC mice, as determined by ELISA (n=5) in ng mg−1from pancreas. ANOVA was used as statistical test. *P<0.01, **P<0.001. (c) Frequency (Freq.) of metastases (mets) in liver and lung of KPC/control and KPC/BK-1361 mice. (d) IHC of mice at week 12. Representative Periodic Acid Schiffs (PAS) staining in KPC/saline versus KPC/BK-1361 pancreas; scale bar, 200 μm. (e) Whisker plot with quantification of invasive PDAC in saline and BK-1361-treated KPC mice. Tukey-type analysis was used for statistics; **P<0.001 (Student’st-test). (f) Whisker plot of normal acinar area in KPC/saline and KPC/BK-1361-treated pancreata (n=5), Tukey-type analysis, *P<0.05 (Student’st-test). (g,h) PAS staining, ADAM8 and pERK1/2 IHC in KPC/control (g) and KPC/BK-1361 (h) mice. Arrowheads indicate focal acinar cell staining, arrow indicates nuclear staining and asterisks mark identical positions. Note loss of ductal architecture in control versus BK-1361-treated mice with positive staining for ADAM8 and pERK1/2. Quantification of IHC for KPC/saline and KPC/BK-1361 pancreas reveals less staining for pERK1/2 in BK-1361 versus saline-treated pancreata. Tukey-type statistical analysis was performed. **<P<0.001 (Student’st-test). Scale bar ind, 100 μm. Figure 7: Application of peptide BK-1361 in PDAC mice. ( a ) Kaplan–Meier analysis of KPC/saline, KPC/BK-1362 (CP) and KPC/BK-1361 mice ( n =10 in each group). Median survival times (MSTs) are given in the diagram; statistical analysis was carried out using a log-rank test with P <0.001. ( b ) Concentration of soluble ADAM8 (sADAM8) in normal mouse pancreas (wt) and in pancreata of saline-treated and BK-1361-treated KPC mice, as determined by ELISA ( n =5) in ng mg −1 from pancreas. ANOVA was used as statistical test. * P <0.01, ** P <0.001. ( c ) Frequency (Freq.) of metastases (mets) in liver and lung of KPC/control and KPC/BK-1361 mice. ( d ) IHC of mice at week 12. Representative Periodic Acid Schiffs (PAS) staining in KPC/saline versus KPC/BK-1361 pancreas; scale bar, 200 μm. ( e ) Whisker plot with quantification of invasive PDAC in saline and BK-1361-treated KPC mice. Tukey-type analysis was used for statistics; ** P <0.001 (Student’s t -test). ( f ) Whisker plot of normal acinar area in KPC/saline and KPC/BK-1361-treated pancreata ( n =5), Tukey-type analysis, * P <0.05 (Student’s t -test). ( g , h ) PAS staining, ADAM8 and pERK1/2 IHC in KPC/control ( g ) and KPC/BK-1361 ( h ) mice. Arrowheads indicate focal acinar cell staining, arrow indicates nuclear staining and asterisks mark identical positions. Note loss of ductal architecture in control versus BK-1361-treated mice with positive staining for ADAM8 and pERK1/2. Quantification of IHC for KPC/saline and KPC/BK-1361 pancreas reveals less staining for pERK1/2 in BK-1361 versus saline-treated pancreata. Tukey-type statistical analysis was performed. **< P <0.001 (Student’s t -test). Scale bar in d , 100 μm. Full size image Our study links the available clinical data on ADAM8 expression in pancreatic cancer cell lines and in PDAC [15] to mechanistic data on ADAM8 in PDAC tumour progression. Using a novel proof-of-concept ADAM8 inhibitor, we demonstrate that ADAM8 inhibition in PDAC leads to reduction of tumour load, infiltration and metastasis in vivo by affecting downstream signalling of ADAM8, thus further supporting the important role of ADAM8 in PDAC. ERK1/2 signalling is considered a major pathway in PDAC, and the EGF/EGFR pathway has been established as an upstream effector of ERK1/2, so that PDAC development and progression is associated with overexpression of EGFR ligands and ADAM17 (refs 43 , 44 ). Aberrant EGF signalling is associated with ERK1/2 signalling in tumour proliferation and migration of pancreatic cancer cells [45] . Since ADAM8 is an active shedding enzyme, evidence of a function of ADAM8 in EGF/EGFR signalling was investigated. No ADAM8-dependent shedding of EGFR ligands such as EGF, epiregulin, amphiregulin and HB-EGF was detected in substrate screens ( Supplementary Fig. 8 ). This suggests that ADAM8 could act independent from the EGF/EGFR pathway, as demonstrated for ADAM10 and ADAM17 (ref. 14 ). Thus, it is likely that ADAM8 stimulates non-EGFR pathways for PDAC progression, which is in agreement with recent experimental observations that progression of PDAC is beyond sole EGF function [46] . For this hypothesis, we provide experimental evidence by demonstrating a link between ADAM8 and ERK1/2 signalling. Our data suggest that ADAM8 interacts with β1 integrin, an essential signalling module in PDAC [47] . The β1-associated signalling pathways involving kinases such as FAK, p38, Akt and ERK1/2 are altered by expression of ADAM8. In particular, ERK1/2 activation is correlated with ADAM8 levels, as shown for cells either overexpressing ADAM8 or AsPC-1 cells bearing a genetic ADAM8 knockdown. In accordance with potent effects of ERK1/2 inhibitors PD98059 and U0126 on reducing Panc1 cell invasion, we propose an ADAM8-induced ERK1/2 activation via the ADAM8 cytoplasmic domain, thereby regulating MMP activities more effectively than inhibitors for Akt and p38. Although ADAM8 can cleave fibronectin [12] , the effect of ADAM8 on cell migration into different ECM substrates could better be explained by ERK1/2 activation in Panc1 cells that regulates the extracellular activities of MMPs. In accordance, increased extracellular activities of MMP-2 and MMP-14 were detected by PrAMA assays. MMP-2 was shown to promote PDAC significantly [48] , [49] , and MMP-2 inhibitors were exploited in Panc1-derived xenografted tumours, resulting in reduced tumour load [50] . Moreover, the role of MMP-14 has been investigated in PDAC and its role in invasion into collagen I, the most abundant ECM present in human PDAC, and its role in cancer invasion has been demonstrated [8] . MMP-2/ MMP-14 induction, however, was not detected on transcriptional levels ( Supplementary Fig. 4 ). Thus, ADAM8-dependent kinase activation such as FAK and ERK1/2 may increase the release of MMP-2 and MMP-14, respectively. To support this notion, FAK and ERK1/2 were shown to regulate MMP release [51] , [52] . MMP-9 is undetectable in Panc1 cells, so that the effect of FAK and ERK1/2 on MMP release is restricted to MMP-2 and MMP-14, respectively. Their activities are interlinked as pro-MMP-2 activation and MMP-14 processing are concomitant events [53] . Xenograft data demonstrate that ADAM8 causes increased invasiveness and tumour growth in vivo . In cell culture, serum-dependent and -independent growth of Panc1 cells was not affected, suggesting that the observed growth relates to infiltrative growth. It is interesting to note that in the orthotopic PDAC model, non-invasive Panc1 cells (Panc1_ctrl or Panc1_A8 cells in mice treated with BK-1361) showed intratumoral hypoxia and necrosis. Hypoxia stimulates ADAM8 expression in a range of PDAC cell lines and Panc1 cells weakly in culture [54] ; however, our data demonstrated a strong induction of ADAM8 under hypoxic conditions in vivo . It is likely that ADAM8 stimulates angiogenesis under hypoxic conditions, as shown earlier in a model of retinopathy [34] . It is remarkable how significantly ADAM8 contributed to tumour cell invasion and metastasis in the PDAC models. Consistent with a proposed role of ADAM8 in PDAC progression, we performed a chemotherapy study in KPC mice by initiating BK-1361 treatment at the onset of PanINs ~4 weeks of age [2] . Given the high degree of specificity reported for BK-1361 towards ADAM8 (see Table 2 for details), it is likely that BK-1361 has selectivity for ADAM8 over other ADAM proteases. However, since BK-1361 mimics an integrin-binding motif, off-target effects may exist and could act on integrins, in particular on β1 integrin. In this respect, unwanted side effects of BK-1361 by inhibition of non-tumour cell located in β1 integrin should be excluded. However, our in vivo data in PDAC mice suggest that off-target effects by BK-1361 may not affect the therapeutic benefit, given the prolonged survival of KPC mice treated with BK-1361 (median survival 15.5 weeks for saline versus 24.2 weeks for BK-1361-treated KPC mice). In terms of percentage survival, ADAM8 inhibition in KPC mice was similarly effective as EGFR inhibition by erlotinib/gemcitabine combination therapy [43] , considering the stringency of the PDAC model used. For further clinical trials, a combination therapy might be beneficial with potentially additive effects of an ADAM8 inhibitory and an anti-EGFR therapy. Our in vitro studies demonstrated that ADAM8 activity requires dimer or greater order multimerization. As reported for ADAM12 and ADAM17, complex formation revealed ambiguous results, similar to our observations of ADAM8 dimers and trimers that were detectable in native gels. However, the precise mechanism of higher order aggregate formation remains to be elucidated and a number of domains have been implied in this process [55] , [56] . From the literature, different aggregation mechanisms of domains functionally also present in ADAM8 have been proposed and there may be several modes of interaction [55] , [56] . We hypothesize that these interactions may occur sequentially, as the ADAM8 DI domain interaction, blocked by BK-1361 prevents further complexes from forming. Since we detected dimers and trimers in the native gel at low concentrations of recombinant ADAM8, we interpret these data that dimers are formed by DI domain interactions, whereas trimers could be formed by different interactions involving the EGF-like domain, as a model for ADAM17 multimerization proposes [55] . Indeed, high concentrations of ADAM8 in vitro lead to higher order multimers such as aggregates of two dimers and/or two trimers, thereby suggesting the presence of such interactions apart from the DI domain interactions ( Supplementary Fig. 3e ). Given the effect of BK-1361 on preventing any ADAM8–ADAM8 interactions, we conclude that initial dimer formation is a critical step in ADAM8 multimerization so that all higher aggregates are prevented from forming by BK-1361. For most ADAM family members, modelling of their DI domains revealed a so-called C-fold scaffold [57] that is inaccessible at the position of the IBL, as shown in the X-ray structure for ADAM10 (ref. 41 ). Homology modelling of the ADAM8 DI domain based on ADAM10 structural data reveals that the IBL is significantly shifted towards an extended loop structure as this was shown for ADAM28 (ref. 58 ). Initial proof for the functionality of ADAM8-binding peptides was obtained by blocking homophilic interactions in cell-binding assays [36] with EC 50 values in the low nanomolar range using BK-1361 and derived peptides. Since there is no homologous amino-acid sequence in the IBL of other ADAM proteases, our approach combines the advantage of high specificity with little or no off-target effects as judged by the lack of toxicity of BK-1361. In conjunction with no expected side effects of ADAM8 inhibition as deduced from ADAM8-deficient mice [28] , [29] , ADAM8 inhibition might be an effective therapy option in mouse PDAC that accurately mirrors human pathology. As first-in-class inhibitor, BK-1361 is structurally similar to cilengitide, an α v integrin-binding angiogenesis inhibitor that raised no safety issues in patients, and is orally available but failed in phase III trials owing to unwanted side effects. Even a short in vivo half-life of ~34 min for BK-1361 ( Supplementary Fig. 10 ), comparable to the half-life of cilengitide, should not limit the therapeutic use of BK-1361, and thereby provides a platform for further preclinical studies including alternative delivery routes and structure-activity relationship. Mice Kras LSL −G12D ; Trp53 R172H/+ ; Pdx Cre/+ (KPC) were described earlier [2] . After weaning, all mice were genotyped. Equal numbers of male and female mice were taken for analysis. All animal experiments were conducted in accordance with Home Office regulations under a relevant project licence (T.H.) and with the German Law on the protection of animals, and were approved by the Local Government (Regierungspräsidium Giessen, J.W.B.). Cell lines Panc1 and AsPC-1 cells were obtained from Sigma (UK); HEK-293, COS7 and MDA-MB-231 cells were purchased from American Type Culture Collection (ATCC). AsPC-1 cells were grown in RPMI medium; all other cell lines were grown in DMEM (Dulbecco’s-modified Eagle medium, Invitrogen, Groningen, The Netherlands), with all media containing 10% fetal calf serum, 1% penicillin/streptomycin and 1% glutamine (Invitrogen, UK). For all experiments, cells were kept in humidified atmosphere at 37 °C/5% CO 2 . Antibodies Human recombinant ADAM8 ectodomain (1031-AD), recombinant ADAM9, ADAM10 and ADAM17, and MMP-2 and MMP-14, human phospho-MAPK Array Kit (ARY002B) and Proteome Profiler soluble receptor array (ARY012) were obtained from R&D Systems (Abingdon, UK). For simultaneous detection of mouse and human ADAM8, a rabbit polyclonal antibody was purchased from Biorbyt (orb 4376, 1:1,000). For IP and native gel electrophoresis, an antibody against the ectodomain of ADAM8 (R&D Systems, AF1031, 1:1,000) was used, for detection of human ADAM8 in western blots, we used an antibody against the cytoplasmic domain of ADAM8 (AB19017; Millipore, Watford, UK, 1:1,000). MMP-2 (R&D Systems, 1;1,000), MMP-9 (Genetex, Irvine, USA, 1:2,000), MMP-14 (R&D Systems, 1:1,000), Birch pollen profilin (BiPro 4A6, Antibody Facility, Braunschweig University, Germany, 1:2,000) and integrin β1 (sc-8978; Santa Cruz Biotechnology, USA, 1:500). Detection of CD23 was performed using an anti-HA antibody (3F10, Mannheim, Germany, 1:1,000). Antibody 12G10 (Abcam, Cambridge, UK, 1:1,000) was used to detect activated integrin β1. For blocking integrin β1, antibody P4C10 from Millipore (1:500) was used. Specific antibodies against the phosphorylated forms of ERK1/2 (T202/Y204; Cell Signaling, Hitchin, UK, 1:1,000), Akt (Ser473; Cell Signaling, 1:1,000 and Thr308; Cell Signaling, 1:1,000), p38γ (T180/Y182; R&D Systems, 1:1,000), Phophatase and tensin homolog (PTEN) (Ser380, Cell Signaling, 1:1,000), c-Raf (Ser 259, Cell Signaling, 1:1,000), MEK1/2 (Ser217/221, Cell Signaling, 1:1,000) and FAK (Y397; BD Biosciences, Oxford, UK, 1:1,000) were used. Horseradish peroxidase (HRP) conjugates antibodies were purchased from Sigma and Southern Biotech (both UK, 1:2,000) and fluorescently labelled antibodies were obtained from Invitrogen and Abcam (1:1,000). The inhibitor tablets cOmplete w/o EDTA and PhosSTOP were purchased from Roche. Peptides Cyclic peptides (named BK-n) were synthesized by Peptide 2.0 (Canada). Purities were >97%. Peptide identities were verified by high-performance liquid chromatography (HPLC) and mass spectrometry (MS). Fluorescent peptides contain 5-carboxy-fluoresceine (FAM) as fluorophore and Dabcyl ([4-((4-(dimethylamino)phenyl)azo)benzoic acid]) as a quencher [59] . Dinitrophenyl-labelled peptides were purchased from the UNC Chapel Hill peptide synthesis laboratory. Oligonucleotides . Oligonucleotides for PCR and site-directed mutagenesis were synthesized by Sigma. Cloning of ADAM8 constructs Full-length human ADAM8 cDNA was obtained by reverse transcription and PCR (hA8fw 5′- ATGCGCGGCCTCGGGCTCT -3′, hA8Sto.as 5′- CTAGGGTGCTGTGGGAGCTCCG -3′) from AsPC-1 cells. The PCR product was cloned into the expression vector pTarget (Promega) and the sequences of the ADAM8 constructs were verified by DNA sequencing. The C-terminally tagged ADAM8 constructs (EGFP, mCherry and BiPro [36] ) were generated by PCR using cloning primers (hA8SgfI 5′- GAGGCGATCGCCATGCGCGGCCTCGGGCTC -3′, hA8MluI 5′- GCGACGCGTGGGTGCTGTGGGAGCTCC ) and ligated into the pCMV6 expression vector (Origene) using the Mlu I and Sgf I restriction sites, respectively. Transfection experiments LTX Lipofectamine (Invitrogen) was used in cell transfection assays according to the manufacturer’s instructions. Cells were lysed 48 h later in modified RIPA buffer (50 mM HEPES pH 7.4, 150 mM NaCl, 1% NP40, 0.5% sodium deoxycholate, 0.1% SDS, 10 mM 1,10-phenanthroline, cOmplete EDTA free and PhosSTOP) and sonicated. A Bradford assay (Thermo Scientific) was used to determine the protein concentrations in whole-cell lysates and in SNs. Generation of Panc1_A8 cells Panc1 cells were co-transfected with a full-length ADAM8 construct (cloned in pTarget) and the pRFP-C-RS vector (Origene) encoding for red fluorescence protein (RFP). Control cells were transfected with RFP vector only. Twenty-four hours after transfection, cells were treated with the respective selection antibiotics (1 μg ml −1 puromycin and 1 mg ml −1 G418). Resistant RFP-positive cells were isolated by fluorescence-activated cell sorting (FACS). ADAM8 expression in single-cell clones was analysed by western blotting and quantitative reverse transcription PCR. Generation ADAM8 knockdown cells AsPC-1 cells were stably transfected with HuSH sh ADAM8 constructs (TF314948, Origene) with the target sequence 5′- GCGGCACCTGCATGACAACGTACAGCTCA -3′ and selected with puromycin (1 μg ml −1 ). Around 20 cell clones were selected and checked for successful knockdown of ADAM8 . To generate control cell clones, a construct with a scramble shRNA sequence was used. Quantitative PCR analysis After reverse transcription using 1 mg of total RNA, quantitative PCR was performed using SYBR Green kits (Bioline, Luckenwalde, Germany) in a STEP-One Light cycler (ABI Systems, Weiterstadt, Germany). As a housekeeping control gene, acidic ribosomal gene XS13 was used. The primers were as follows: ADAM8 : fw: 5′- ACAATGCAGAGTTCCAGATGC -3′; rev: 5′- GGACCACACGGAAGTTGAGTT -3′; XS13 : 5′- TGGGCAAGAACACCATGATG -3′; rev: 5′- AGTTTCTCCAGAGCTGGGTTGT -3′. ADAM8 ELISA To determine soluble ADAM8 in mouse tissue, a commercial ADAM8 ELISA assay (Hoelzel Diagnostica, Cologne, Germany) was used according to the manufacturer’s instructions. Pancreas tissues were homogenized in 10 volumes of ice-cold PBS containing 1 mM ethylene glycol tetraacetic acid (EGTA) and cOmplete Inhibitor Mix (Roche), clarified by centrifugation (10,000 r.p.m., 10 min at 4 °C). SNs were used for ELISA. In vitro autocatalysis assay with ADAM8 Inactive recombinant human ADAM8 (Met1-Pro497) was obtained from R&D Systems. ADAM8 autocatalytic activation assays were performed in 50 mM Tris, 10 mM CaCl 2 and 150 mM NaCl, pH 7.5 (TCN) buffer for the indicated times at 37 °C. If applicable, peptides were diluted 1:1,000 in the assay. To avoid evaporation during longer incubation periods, the enzyme solutions were overlaid with mineral oil. Native gel electrophoresis To assess complex formation of recombinant pro-ADAM8, native gel electrophoresis was performed. Samples were dissolved in native buffer to retain protein complexes (0.02% β-glycerophosphate, 0.02% sodium orthovanadate, 0.04% EGTA, 0.6% HEPES, 0.03% EDTA, 0.58% sodium chloride, 1.5% dodecyl maltoside and 0.11% sodium pyrophosphate decahydrate; Abcam) with 100 ng pro-ADAM8 in the presence of either 200 nM CP (BK-1362) or BK-1361 were prepared and run on a 4–16% native gel (Novex, Life Technologies, Darmstadt, Germany). As molecular weight marker, Novex Native Mark was used. Gels were blotted and stained with AF1031 (see antibody section). Activity assays with ADAM8 Activity of recombinant ADAM8 catalytic/DI domain was monitored at 2 min intervals using the fluorescent substrate Dabcyl-HGDQMAQKSK(5FAM)-NH 2 (ref. 59 ), emulating the cleavage site of CD23, a physiological substrate for ADAM8 (Fourie et al . [30] ). Assays were performed in a multiwell plate reader (Fluostar Optima, BMG Labtech, Offenburg, Germany) using an excitation wavelength of 485 nm and an emission of 530 nm, with activity expressed as fluorescence units per hour. The substrate concentration was 10 μM in assay buffer (20 mM Tris, pH 8.0, 10 mM CaCl 2 and 6 × 10 −4 % Brij-35). Reactions were run in a 96-well black-coated plate. The concentration of ADAM8 enzyme was typically 10 ng per reaction. For inhibition assays using the cyclic peptide inhibitor, concentrations varied from 10 nM up to 5 μM. Determination of MMP/ADAM activities in PDAC cell lines PrAMA analysis [42] was performed as follows: Panc1, AsPC-1 cells and derivates were cultured in duplicate using a six-well plate for 24 h in serum-free DMEM medium without phenol red. Medium was removed, spun to remove cell fragments and set aside for assaying. Cells were washed with PBS and then scraped from the plate and resuspended in a 1.5-ml tube in a cold solution of 0.25 M sucrose, 50 mM Tris, pH 8, and a protease inhibitor mixture (cOmplete, Roche Applied Science). Cells were broken via pipetting up and down, and the suspension was spun at 13,000 g to pellet the membranes, which were resuspended and washed with sucrose buffer. After pelleting, membranes were resuspended in 200 μl of sucrose buffer per well of cells. Protein concentrations were determined using the Bio-Rad BPA assay. The medium and membrane suspension were tested for MMP/ADAM activity by using the PrAMA analysis technique developed by Miller et al . [41] using substrates PEPDab005, PEPDab010, PEPDab008, PEPDab013 and PEPDab014, which varied in their specificities towards different ADAM family members and MMPs. Briefly, 12.5 μM substrate concentrations in 60 μl of assay buffer (see above) were incubated with either 20 μl of medium or 10 μl of resuspended membranes. Fluorescence units versus time were monitored with a Fluostar BMG Optima using excitation and emission wavelengths of 485 and 530 nM, respectively. Specific protease activities were inferred with PrAMA by comparing the pattern of substrate cleavage rates for each sample to a matrix of known substrate specificities for ADAM8, ADAM10, ADAM17, MMP-2 and MMP-14 that were determined using purified enzymes (Miller et al . [41] ). Before performing PrAMA, substrate cleavage rates were first converted to fold change over control measurements as indicated. Each PrAMA experiment was repeated three times and values for activities are given as relative to defined control measurements (a.u.). Immunofluorescence MDA-MB-231, Panc1 cells and stable derivatives were grown on coverslips, and were fixed with 3.7% paraformaldehyde. ADAM8 was detected in unpermeabilized cells by goat polyclonal antibody AF1031 (R&D Systems) as primary antibody. As secondary antibody, we used goat-anti-rabbit-Cy3 (1:500, Sigma). Images were acquired by confocal microscopy imaging using a Nikon A1R microscope equipped with CFI Plan Fluor × 40 oil objective. Images were captured and exported with NIS Elements software (Nikon) and presented as TIF files. Immunoblotting and IP experiment Equal amounts of protein were loaded onto 10% reducing polyacrylamide (PAA) gels. The proteins were transferred on nitrocellulose, unspecific binding sites were blocked (5% skimmed milk, 0.1% Tween-20 in PBS) and specific antibodies were used to detect the proteins of interest. An enhanced chemiluminescent (ECL) substrate (Thermo Scientific) for HRP enzyme and a chemiluminescence reader (Intas, Goettingen, Germany) were used for visualization. Images in Figs 4 and 5 have been cropped for presentation. Full size images are presented in Supplementary Figs 11 and 12 . For IP assays, the cells were lysed in co-IP buffer (50 mM HEPES pH 7.4, 150 mM NaCl 2 , 1% NP40, 0,5% sodium deoxycholate, 1,5 mM MgCl 2 and cOmplete). The sonicated lysates were centrifuged two times at full speed to remove cell debris. Cleared lysates were subjected to IP using specific antibodies in concentrations of 0.2 μg ml −1 (for anti-BiPro) and 2.5 μg ml −1 (for anti-ADAM8) overnight at 4 °C. As unspecific binding controls, IgG was used instead of specific antibodies. After binding of precipitated material to Protein-G-sepharose and washing steps, the precipitated proteins were eluted by boiling in 2 × SDS-loading buffer and were analysed by western blotting. Gelatine zymography Protein samples were prepared in non-reducing sample buffer without boiling before the experiment. Gelatin (0.1%) was added in a separating gel to co-polymerize with PAA. During electrophoresis, proteins are separated in the PAA gel, while SDS present in the gel preserves MMPs in an inactive state. After the run, gels were washed with renaturing buffer (2.5% Triton X-100; 2 × 30 min each) that resulted in partially renatured MMPs with restored activity. The gel was incubated in developing buffer (50 mM Tris, pH 7.5, 200 mM NaCl, 4 mM CaCl 2 and 0.02% Brij-35; 30 min at RT, followed by 24 h at 37 °C in fresh developing buffer). Next day, the gel was dyed in Coomassie staining buffer for 1 h followed by Coomassie destaining solution to visualize bands of active enzyme. FRET/FLIM FLIM was performed and data were analysed as described previously [60] . FLIM capability was provided by time-correlated single-photon counting electronics (Becker & Hickl, SPC 700). Widefield acceptor monomeric Red Fluorescent protein (mRFP) images were acquired using a CCD camera (Hamamatsu) at exposure times of <100 ms. Data were analysed using TRI2 software (developed by Dr Paul Barber). All histogram data are plotted as mean FRET efficiency from >12 cells per sample. Lifetime images of exemplary cells are presented using a pseudocolour scale whereby blue depicts normal GFP lifetime (that is, no FRET) and red depicts reduced GFP lifetime (areas of FRET). Each experiment was repeated at least three times. Analysis of variance (ANOVA) was used to test statistical significance between different populations of data. Activated MAPK assay The human phospho-MAPK Array Kit (ARY002B; R&D Systems) was used to analyse the influence of ADAM8 on the activation state of altogether 26 MAPKs and other serine/threonine kinases. The assay was used according to the manufacturer’s instructions. In brief, cells of the stable control PANC1 clone and the ADAM8 overexpressing clone were lysed in lysis buffer 6, sonicated and a Bradford assay was used to determine the protein concentrations. Each array membrane was incubated in 2 ml array buffer 5 for 1 h at room temperature on a rocker. An amount of 1 mg of each lysate was mixed with array buffer 1 to a final volume of 1.5 ml. A volume of 20 μl reconstituted Detection Antibody Cocktail was added and the mixture was incubated for 1 h at room temperature. After removal of array buffer 5 from the membranes, the lysate Detection Antibody mixture was added to the membrane. The membranes were incubated at 4 °C on a rocker overnight. Each membrane was washed three times with 1 × wash buffer (20 ml, 10 min each) and incubated with 2 ml streptavidin-HRP (1:2,000 in array buffer 5) for 30 min at room temperature on a rocker. After three repeating washing steps with 1 × wash buffer (20 ml, 10 min each), an ECL substrate (Thermo Scientific) for HRP enzyme and an ECL camera (Intas, Goettingen, Germany) were used to detect the signals. The signals were quantified with the National Institutes of Health (NIH) ImageJ software package (freeware). ADAM8 DI structure modelling A BLAST (a) search of the Protein Data Bank (b) using the ADAM8 sequence revealed the top structure hits as Russell’s viper venom metalloproteinase (2e3x) (c) and vascular apoptosis-inducing protein-2 (2ero) (d). 2E3X and 2ERO align structurally at 2.33 Å using the alignment in Supplementary Fig. 1 . The structure of ADAM10 (2AO7) (e) was also aligned even though it was eighteenth in the BLAST results. The per cent identity matrix is shown in Supplementary Fig. 2 . Administration of cyclic peptide BK-1361 in mice Lyophilized cyclic peptide was dissolved in sterile PBS to a concentration of 1 μg μl −1 . Since neither an acute (single injection) nor a chronic toxicity (repeated weekly injections over a total of 4 weeks) using a dosage of 10 μg g −1 body weight via intraperitoneal route was observed based on organ histology after necropsy ( Supplementary Fig. 9 ), this dosage regimen was administered throughout the experiments presented in this study. Equal volumes of sterile PBS were injected as control. For KPC mice, BK-1361 injections were started at 4 weeks of age and continued for over 8 weeks. Mice were constantly monitored and were killed when they reached end point criteria. Orthotopic injections Orthotopic pancreatic cancer tumours were implanted into 6-week-old female CD1 nu/nu mice. Ketamine/xylazine (100/10 mg kg −1 ) was used for anaesthesia. The left side of the mouse was shaved and the fur was completely removed. The surgical area was sterilized with an iodine solution (Povidone-iodine, Novaplus, Irving, TX, USA) and a small incision (<1 cm) was made through the skin and abdominal wall at the base of the spleen. The spleen was gently pulled through the incision, exposing the tail of the pancreas. The cell-Matrigel solution (1 × 10 6 cells in 50 μl) was injected into the tail of the pancreas. The Matrigel was allowed to set (~ 10 s), the needle was gently removed from the pancreas and the area was swabbed with iodine to devitalize any stray cells in the injection site. The pancreas and spleen were replaced in the abdomen and the incision site closed with 3–4 sutures (Ethilon 5–0 PS-3, Ethicon, Piscataway, NJ, USA). The Matrigel method of orthotopic tumour implantation has resulted in 100% tumour uptake with little evidence of extra-pancreatic leakage. Panc1 and AsPC-1 cell-derived tumours were analysed 12 days after implantation. Statistical analysis Invasion assays and western blot data were analysed by one-way ANOVA. For in vivo experiments, two-way ANOVA using Shapiro–Wilk normality was used. For pairwise comparisons of tumour weights/volumes and tissue pathologies (acinar tissue and infiltration rates), including ImageJ analyses, Tukey-type linear contrast tests were used. Survival was estimated as a Kaplan–Meier survival curve, and the statistical analysis was carried out using a log-rank test for the censored data. Based on the obtained results, the data were considered not significant ( P ≥0.05), significant * ( P ≤0.05), highly significant ** ( P ≤0.01) or very highly significant *** ( P ≤0.001). How to cite this article: Schlomann, U. et al . ADAM8 as a drug target in pancreatic cancer. Nat. Commun. 6:6175 doi: 10.1038/ncomms7175 (2015).